Potential regime shift in decreased sea ice production after the Mertz Glacier calving Variability in dense shelf water formation can potentially impact Antarctic Bottom Water (AABW) production, a vital component of the global climate system. In East Antarctica, the George V Land polynya system (142–150°E) is structured by the local 'icescape', promoting sea ice formation that is driven by the offshore wind regime. Here we present the first observations of this region after the repositioning of a large iceberg (B9B) precipitated the calving of the Mertz Glacier Tongue in 2010. Using satellite data, we find that the total sea ice production for the region in 2010 and 2011 was 144 and 134 km 3 , respectively, representing a 14–20% decrease from a value of 168 km 3 averaged from 2000–2009. This abrupt change to the regional icescape could result in decreased polynya activity, sea ice production, and ultimately the dense shelf water export and AABW production from this region for the coming decades. Antarctic Bottom Water (AABW) is a critical component of the global climate system [1] , [2] , occupying the abyssal layer of the World Ocean and driving the lower limb of the global meridional circulation. In East Antarctica, the local source of AABW to the Australian–Antarctic Basin is the dense shelf water exported from the George V Land coast [3] , [4] , [5] , [6] ( Fig. 1 ). Observations of the George V Land (hereinafter GV) continental shelf from 1999–2004 describe a dual system of dense shelf water formation from enhanced sea ice production in the polynyas over the Adélie and Mertz Depressions [7] , [8] , [9] . An important feature of the GV regional icescape (that is, the interaction of topography, ice sheet/ice shelf configuration and fast ice) has been the blocking of the westward advection of sea ice [10] , [11] , [12] by the existence of the Mertz Glacier Tongue (MGT), together with a large iceberg (B9B) and surrounding fast ice. This promotes polynya activity, and hence dense shelf water formation, which is driven by cold offshore winds [13] , [14] . In the Adélie Depression, polynyas typically formed in the coastal bays (Commonwealth, Watt and Buchanan Bays labelled CB, WB and BB, respectively) and along the western lee of the MGT. In the Mertz Depression, a smaller polynya formed in the western lee of the grounded iceberg B9B, which moved into the region from the Ross Sea in 1992 [10] . Both the MGT and B9B have had fast ice extensions (sometimes referred to as 'daggers'), which formed each winter around the grounded icebergs to their north and contributed to the respective polynya zones ( Fig. 2a ). 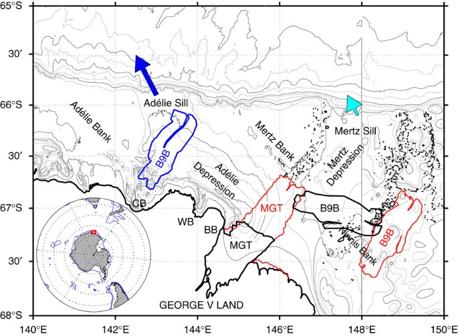Figure 1: The George V Land region. Map following ref16. Major features are as named and include the Adélie (and Mertz) Depression, Sill and Bank and Ninnis Bank. CB, WB and BB are as indicated. Reported pre-calving outflow regions of dense shelf waters capable of producing AABW from the two depressions indicated by the blue arrows9. Key icescape features include the pre- (red) and post-calving positions of the MGT (black) and iceberg B9B (2010: black and 2011: blue). Black scattered dots indicate grounded icebergs. Inset: George V Land in East Antarctica. Figure 1: The George V Land region. Map following ref 16 . Major features are as named and include the Adélie (and Mertz) Depression, Sill and Bank and Ninnis Bank. CB, WB and BB are as indicated. Reported pre-calving outflow regions of dense shelf waters capable of producing AABW from the two depressions indicated by the blue arrows [9] . Key icescape features include the pre- (red) and post-calving positions of the MGT (black) and iceberg B9B (2010: black and 2011: blue). Black scattered dots indicate grounded icebergs. Inset: George V Land in East Antarctica. 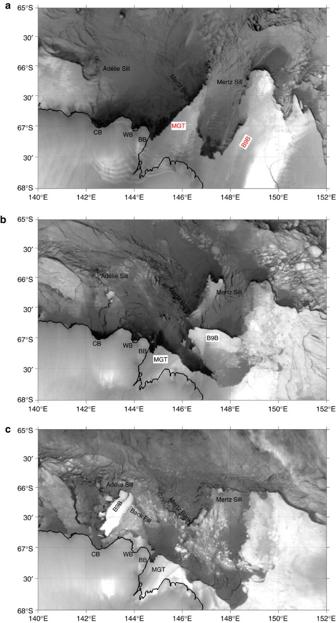Figure 2: Regional icescapes. MODIS satellite imagery showing the structural changes to the GV polynya system before and after the MGT calving. (a–c) correspond to the pre-calving (19 July 2006) and post-calving (11 June 2010 and 31 July 2011) winter polynya regimes, respectively. Full size image Figure 2: Regional icescapes. MODIS satellite imagery showing the structural changes to the GV polynya system before and after the MGT calving. ( a–c ) correspond to the pre-calving (19 July 2006) and post-calving (11 June 2010 and 31 July 2011) winter polynya regimes, respectively. Full size image In early 2010, the repositioning of iceberg B9B parallel to the coast over the Ninnis Bank precipitated the calving of the MGT [15] , with newly formed iceberg C28 departing the region shortly thereafter ( Fig. 2b , hereinafter referred to as 'post-calving-2010'). In 2011, B9B migrated across the Adélie Depression and regrounded in Commonwealth Bay with a NNE-ward orientation ( Fig. 2c , hereinafter referred to as 'post-calving-2011'). Numerical ocean-ice model simulations [16] suggest that the ocean circulation and sea ice production in the region changes immediately after the calving, resulting in a decrease (up to 23%) in dense shelf water export. This study is the first observational assessment of the change in the GV region after the MGT calving. Sea ice production estimates are presented using a thin ice thickness algorithm based on satellite Special Sensor Microwave/Imager (SSM/I) data and a heat flux calculation [17] , [18] , [19] , in conjunction with a fast ice time series and climatology derived from NASA moderate resolution imaging spectroradiometer (MODIS) satellite imagery [20] . We examine the change in sea ice production in 2010 and 2011, relative to the mean annual sea ice production over the preceding years from 2000–2009. Using a simple statistical model, we discuss the post-calving sea ice production results with respect to the interannual variability of pre-calving sea ice production and its relationship with the atmospheric forcing from ERA-Interim. Spatial distribution of sea ice production The spatial distribution of annual sea ice production (m a −1 ) is shown in Fig. 3 for three scenarios: (a) 'pre-calving', that is, the mean over the period 2000–2009, (b) 'post-calving-2010' and (c) 'post-calving-2011'. The fast ice extent, averaged over the winter months (JJA, red line), is also shown in each case. For the pre-calving case ( Fig. 3a ), the dual system of polynya/dense shelf water formation over the Adélie and Mertz Depressions described earlier is evident east and west of the MGT. Pre-calving, the peak production rates over the Adélie Depression (up to 19 m a −1 ) occurred in the western lee of the MGT and fast ice extension over the grounded bergs to the north (hereinafter referred to as the Mertz Glacier polynya region), as well as in the coastal bays to the west. Similarly, the sea ice production over the Mertz Depression occurred in the western lee of iceberg B9B and the fast ice extension to its north, but with smaller magnitude (up to 8 m a −1 ). This pre-calving regime agrees with the sea ice conditions suggested from the MODIS image in Fig. 2a and is representative of all years from 2000–2009 ( Supplementary Fig. S1 ). The mean total annual sea ice production for 2000–2009 was 168 km 3 . 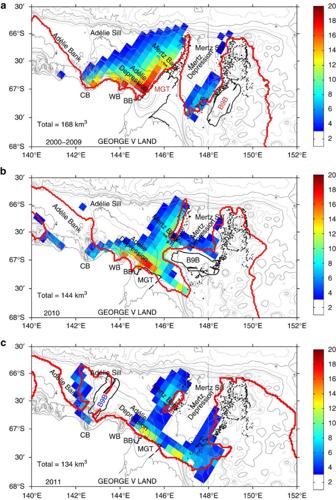Figure 3: Sea ice production. Spatial distribution of cumulative sea ice production (m a−1) is averaged over the freezing seasons (March–October) for (a) 2000–2009, (b) 2010 and (c) 2011. Data are calculated using ERA-Interim data for the total GV polynya system. The maximum fast ice extent is shown from the mean 20-day data over JJA (red line). Figure 3: Sea ice production. Spatial distribution of cumulative sea ice production (m a −1 ) is averaged over the freezing seasons (March–October) for ( a ) 2000–2009, ( b ) 2010 and ( c ) 2011. Data are calculated using ERA-Interim data for the total GV polynya system. The maximum fast ice extent is shown from the mean 20-day data over JJA (red line). Full size image Post-calving in 2010 The post-calving maps in 2010 and 2011 ( Fig. 3b,c ) show significant changes to the distribution and magnitude of sea ice production across the region. In 2010, the peak production occurs along the coast from Watt Bay, across the new front of the Mertz Glacier and as far east as 146°E. The previous Mertz Glacier polynya region still exists from the MGT to the grounded bergs east of the Mertz Bank, assisted by the rotated position of B9B. Reduced production over the Adélie Depression is partially compensated by the new production over the area formerly occupied by the MGT. Production over the Mertz Depression is now divided by the temporary position of B9B with a new zone to the south of the Ninnis Bank from 146–147°E. Overall, the mean total sea ice production for 2010 was 144 km 3 , representing a ∼ 14% decrease from the 2000–2009 mean. B9B in Commonwealth Bay in 2011 The icescape changed again in 2011, this time as a result of the migration of B9B ( Fig. 3c ). B9B generated a new but relatively weak polynya region extending north along the eastern flank of the Adélie Bank from Commonwealth Bay to the shelf break. Production decreased in the Mertz Glacier polynya region, in particular to the south from Watt Bay across the new front of the MGT. This is most likely due to the impact of B9B's migration between 2010 and 2011, and its new location restricting the advection of sea ice away from the Mertz Glacier polynya region ( Fig. 2c ). Conversely, the removal of B9B from its 2010 position could have allowed greater advection of sea ice away from the region to the east, resulting in the new polynya region extending north from 148°E that links up with the previous Mertz Depression polynya. Though there has been a net decrease in sea ice production since the calving, regionally the changes are mixed with some new regions of enhanced sea ice production. We estimate the total sea ice production to be 134 km 3 , representing a further decrease from 2010 and a ∼ 20% decrease from the 2000–2009 mean. Abrupt change versus interannual variability Our key finding that total sea ice production decreased following the calving of the MGT in 2010 agrees with the ocean-ice model simulations by ref. 16 . To examine the significance of these decreases relative to the strong interannual variability reported for the region [11] , [21] , we present the full time series of total sea ice production for the periods 2000–2011 (using MODIS derived fast ice data) and 1992–2010 (using SSM/I derived fast ice data) in Fig. 4 (see also Supplementary Fig. S2 and Supplementary Table S1 for details of the statistical analysis). The interannual variability reflected in the MODIS time series puts into context the post-calving decrease from 2009 to 2010, because it is of a similar magnitude to the decrease from 2003–2004, and the minima in 2010 and 2011 are equivalent to the other peak minima across the period in 2000 and 2004. Using the longer time series with SSM/I fast ice estimates, the 2010–2011 minima in sea ice production remains at the lower limit of the extended sea ice production time series dating back to 1992. We now seek to assess the impact of the structural changes to the icescape on the post-calving decreases in total sea ice production relative to the meteorological driving factors. 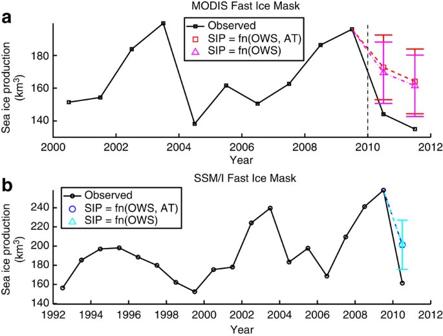Figure 4: Interannual variability and change. The time series of total (Mar–Oct) sea ice production (km3) for the total GV polynya system (seeSupplementary Fig. S1for the actual area) is shown for (a) 2000–2011 (MODIS period) and (b) 1992–2010 (SMM/I period). Predicted sea ice production from statistical regression analysis of OWS and AT, and OWS only is shown for 2010–2011 (red and magenta lines) and 2010 (blue and cyan lines), respectively. Figure 4: Interannual variability and change. The time series of total (Mar–Oct) sea ice production (km 3 ) for the total GV polynya system (see Supplementary Fig. S1 for the actual area) is shown for ( a ) 2000–2011 (MODIS period) and ( b ) 1992–2010 (SMM/I period). Predicted sea ice production from statistical regression analysis of OWS and AT, and OWS only is shown for 2010–2011 (red and magenta lines) and 2010 (blue and cyan lines), respectively. Full size image Applying multiple linear regression to form simple predictive models for total sea ice production, based on predictor variables of offshore wind speed (OWS) and air temperature (AT), we find that the observed decrease in total sea ice production in 2010 and 2011 (MODIS only) relative to 2009 was ∼ 50% greater than the predicted values (red/magenta and blue/cyan points in Fig. 4 ). Additionally, the observed changes lie outside the predicted s.d. of the error. Given that both 2010 and 2011 had strong environmental forcing anomalies favouring sea ice production, that is, cold AT and elevated OWS, relative to the 1992–2011 mean ( Supplementary Fig. S2 ), we speculate that the observed decreases could have been even greater with the reduced OWS and/or warmer AT typical of many previous years. We have no means to account for wind speed in our estimates, but by introducing a 2.25–1.85 K increase in AT, we speculate that the post-calving production in 2010 and 2011 could have been 10–15% lower at 123 and 117 km 3 , respectively. Since the calving of the MGT in early 2010, the GV polynya regime has been in a state of structural transition relating to abrupt changes in the regional icescape. Here, we have shown that in 2010 and 2011 there was a 14–20% reduction in total sea ice production relative to the pre-calving mean. We speculate that ∼ 50% of the decrease in sea ice production in both years can be attributed to the changes in icescape, and that given the known variability in environmental forcing there could be even greater decreases with the current icescape into the future. Currently, B9B is breaking up and after it departs the GV region, we expect that sea ice production could remain below the pre-calving levels until the MGT extension forms again at a mean annual rate of ∼ 1 km a −1 (ref. 15 ). Our observed changes in sea ice production confirm the initial prediction from ocean-ice model simulations of the post-calving regime [16] . These simulations showed that the calving of the MGT had a significant impact on dense shelf water export from this region and subsequent production of AABW to the Australian–Antarctic Basin. Furthermore, a new study of ship-based CTD measurements in the summers of 2008 and 2011 reports a ∼ 0.05 decrease in shelf water salinity since the MGT calving (personal communication Steve Rintoul). This decrease is equivalent to the long-term freshening of dense shelf water ( ∼ 0.01 dec −1 ) in the Adélie Depression since 1950 (not shown) that is similar but weaker to that reported in the Ross [22] and Weddell [23] sectors. The source of this GV freshening has not been confirmed, with no evidence in the available observations to suggest a long-term decrease in sea ice production/brine rejection and/or increase in Mertz Glacier melting. Given the attribution of freshening in the Ross Sea ( ∼ 0.01 dec −1 ) to upstream melting in the Amundsen Sea [22] , then the GV freshening may be influenced by similar mechanism from the Cook Ice Shelf. This abrupt decrease of post-calving effectively doubles the long-term trend to >0.02 dec −1 over length scales incorporating the glacial calving cycle. Under a warming climate scenario, we might expect both the long-term freshening and abrupt changes due to the dynamic ice front to increase. However, the impact of the dynamic ice front is complex and we note that a calved iceberg can increase polynya activity downstream of its grounded location, as B9B did after leaving the Ross Ice Shelf and migrating to the GV region. Our findings present an ongoing challenge to the polar climate modelling community in terms of how to include dynamic ice front changes, such as those currently occurring in the GV region, into simulations of past and future sea ice production, dense shelf water formation and AABW production over multi-decadal timescales. A similar challenge also exists for observational studies attempting to assess long-term climate trends over timescales interspersed with these structural changes to the system. Sea ice production The sea ice production estimation in this study follows |ref. 19 . For the period of 1992–2008 and 2007–2011, F-13 85-GHz and F-17 91-GHz SSM/I data are used, respectively. The bias between the 85-GHz and 91-GHz polarization ratio (PR 85 and PR 91 ) is much smaller ( Supplementary Fig. S3 ) than the error of the ice thickness algorithm ( ∼ 5 cm) [17] . For the periods 1992–2010 and 2000–2011, this study uses fast ice and iceberg mapping from SSM/I [17] and MODIS [20] data, respectively. Our heat flux calculation uses the European Centre for Medium-Range Weather Forecasts Re-Analysis data (ERA-Interim) and the National Centers for Environmental Prediction/Department of Energy Re-Analysis data (NCEP2). Sea ice production is assumed to occur only in the thin ice area where heat flux is negative during March–October [18] . Thus, the November–February production is removed from our sea ice production values (except in the monthly variability figures). We have confirmed that there is little difference in ice production calculated from F-13 85-GHz and F-17 91-GHz data ( Supplementary Fig. S4a ). Quality-controlled SSM/I data are available only until August 2011. For the period from March to August 2011, we compared sea ice production calculated both from preliminary and quality-controlled data, and calculated the bias between the two ( Supplementary Fig. S4b ). For the 2011 sea ice production, we use the value calculated from preliminary SSM/I data with adding of this bias. Although Advanced Microwave Scanning Radiometer-EOS (AMSR-E) data are available at a higher spatial resolution, they are available only from 2003 to 2011 (halted on 4 October 2011). Therefore, the longest continuous record of sea ice production and interannual variability comes from the SSM/I dataset. Fast ice extent The 2000–2011 fast ice time series follows ref. 24 . The detection algorithm generates cloud-free composite images of the surface over 20-day intervals using the MODIS satellite instrument. A modified MODIS cloud mask is used to construct these cloud-free 20-day composite images [25] . During this interval, pack ice becomes smoothed owing to motion, while the fast ice edge remains sharply defined. To overcome problems associated with imperfect cloud masking, a new algorithm was developed and applied to the latter years (2009–2011). This algorithm performs edge detection on non-cloud-masked MODIS granules. Fast ice is identified after assuming that persistent edges represent either the fast ice edge or the coastline (the location of cloud is dynamic, giving no persistent edges). How to cite this article: Tamura, T. et al . Potential regime shift in decreased sea ice production after the Mertz Glacier calving. Nat. Commun. 3:826 doi: 10.1038/ncomms1820 (2012).